Construction of stabilized bulk-nano interfaces for highly promoted inverse CeO2/Cu catalyst As the water-gas shift (WGS) reaction serves as a crucial industrial process, strategies for developing robust WGS catalysts are highly desiderated. Here we report the construction of stabilized bulk-nano interfaces to fabricate highly efficient copper-ceria catalyst for the WGS reaction. With an in-situ structural transformation, small CeO 2 nanoparticles (2–3 nm) are stabilized on bulk Cu to form abundant CeO 2 -Cu interfaces, which maintain well-dispersed under reaction conditions. This inverse CeO 2 /Cu catalyst shows excellent WGS performances, of which the activity is 5 times higher than other reported Cu catalysts. Long-term stability is also very solid under harsh conditions. Mechanistic study illustrates that for the inverse CeO 2 /Cu catalyst, superb capability of H 2 O dissociation and CO oxidation facilitates WGS process via the combination of associative and redox mechanisms. This work paves a way to fabricate robust catalysts by combining the advantages of bulk and nano-sized catalysts. Catalysts with such inverse configurations show great potential in practical WGS applications. Bulk catalysts with stable structure have been applied to many industrial procedures, such as fused Fe for ammonia synthesis [1] and Cu–Zn–Al for water–gas shift (WGS) reaction [2] . In recent years, the introduction of nanotechnology has brought valuable insights into heterogeneous catalysis. Remarkable catalytic performances in many reactions have been discovered for supported nanoparticles, clusters, and single atoms [3] , [4] , [5] , [6] , [7] , of which defects and vacancies on the oxide supports are often considered as important anchoring sites. One major shortcoming of these supported catalysts is the vulnerability against sintering [8] , [9] , [10] . The highly dispersed active sites tend to aggregate and deactivate under reaction conditions. Thus, combining the advantages of bulk and nano-sized catalysts is of great significance, though it seems tough, since the bulk structure contradicts the high dispersion. WGS (CO + H 2 O = CO 2 + H 2 ) reaction is a crucial process in H 2 production industry [11] , to which Cu-based catalysts have been applied for decades [12] , [13] , [14] . Cu–CeO 2 has been considered as promising alternative to Cu–Zn–Al catalyst, while it still suffers from low activity caused by Cu sintering [15] , [16] , [17] . It has been known that the metal–oxide interface plays a critical role in catalyzing WGS reaction, of which the key is the adsorption and activation of reactants [18] , [19] , [20] . To deeply understand the interface effect, catalysts with inverse configuration have been designed [21] , [22] , [23] . Different to commonly supported catalysts, for which active metals are loaded onto the oxide supports, active metals serve as the support for oxides nanoparticles in inverse catalyst [24] , [25] , [26] , [27] . Model inverse CeO x /Cu(111) has shown superior WGS activity to normal Cu/CeO 2 (111), owing to enhanced reducibility of CeO 2 [28] . Meanwhile, the CeO 2 –Cu interface could be highly stable, since bulk Cu has grown well and CeO 2 nanoparticles are anti-sintering under WGS conditions, which is very beneficial to the catalyst stability. Thus, prominent activity and stability promotion of Cu–CeO 2 catalyst is expected by applying inverse configuration. However, the assumed high WGS activity has never been found on real CeO 2 /Cu catalyst, due to severe separation of bulk Cu and CeO 2 nanoparticles [29] . Therefore, strategies to fabricate inverse CeO 2 /Cu catalyst with sufficient bulk–nano interfaces are in great need. Herein, we have constructed stabilized bulk–nano interfaces to fabricate inverse CeO 2 /Cu catalyst, through which the advantages of bulk and nano-sized catalysts are perfectly combined. With an in situ structural transformation, CeO 2 nanoparticles (2–3 nm) are dispersed on bulk Cu, forming sufficient CeO 2 –Cu interfaces with great stability. Enrichment of stable bulk–nano interfaces results in great promotion of WGS activity and stability. The inverse CeO 2 /Cu catalyst achieves a remarkable WGS reaction rate of 47.3 μmol g −1 s −1 (300 °C), which is at least five times of that for other Cu catalysts. Mechanistic study demonstrates the CeO 2 /Cu catalyst possesses superb capability of H 2 O dissociation and CO oxidation, which facilitates WGS reaction via the combination of associative and redox mechanism. Development of such inverse catalyst is very likely to make huge breakthrough in the exploration of other robust catalysts. Catalytic performances of the inverse CeO 2 /Cu catalyst A series of catalysts with different Cu/Ce ratio was prepared via an aerosol-spray method [30] , [31] , [32] . As shown in Supplementary Fig. 1a and c , the inverse CeO 2 /Cu catalyst with Cu/Ce ratio of 9:1 showed the highest and repeatable WGS activity. Increased or decreased proportion of Cu led to lower CO conversion (Supplementary Fig. 1b ). 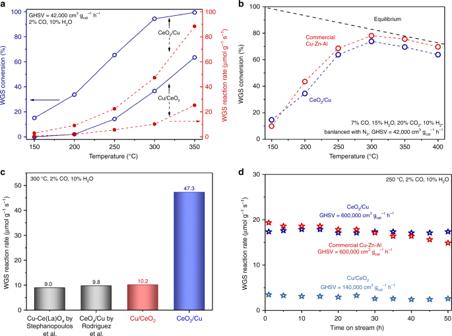Fig. 1 Catalytic performances of the inverse CeO2/Cu catalyst.aWater–gas shift (WGS) activities of the inverse CeO2/Cu and normal Cu/CeO2catalysts.bWGS activities of the inverse CeO2/Cu catalyst and commercial Cu–Zn–Al under industrial atmosphere.cComparison of WGS reaction rates for different catalysts at 300 °C.dTime-on-stream tests of the inverse CeO2/Cu, normal Cu/CeO2catalysts, and commercial Cu–Zn–Al The physical and chemical properties of the catalysts are listed in Supplementary Table 1 . Fresh CeO 2 /Cu catalyst contained 61.5 wt% of Cu, and the Cu content elevated to 82.9 wt% after WGS reaction, due to the reduction of CuO to Cu. The 17.1 wt% CeO 2 loading corresponded well to the finding of Rodriguez et al. [24] , illustrating the optimal CeO 2 coverage on Cu surface was around 20%. For supported Cu/CeO 2 catalyst, 10 wt% of Cu has often been applied to obtain an effective catalyst [33] , [34] , [35] . Therefore, normal Cu/CeO 2 catalyst, with 10.7 wt% of Cu, was chosen for comparison. In Table 1 , the two fresh catalysts exhibited similar specific BET surface areas ( S BET , 46‒48 m 2 g −1 ). After catalysis, the S BET of CeO 2 /Cu catalyst (16.2 m 2 g −1 ) apparently decreased, while that of Cu/CeO 2 catalyst (42.8 m 2 g −1 ) was well preserved. Cu surface area ( S Cu ) was also calculated for both catalysts (see Supplementary Methods for detail). The S Cu of Cu/CeO 2 (71.7 m 2 g −1 ) was also higher than that of CeO 2 /Cu (50.7 m 2 g −1 ). However, the inverse CeO 2 /Cu catalyst exhibited much higher WGS conversion than that of Cu/CeO 2 catalyst (Fig. 1a ). Within the tested temperature range, the reaction rate ( r ) of CeO 2 /Cu measured under kinetics conditions was 4–5 times higher than that of Cu/CeO 2 catalyst. Under the industrial WGS atmosphere, as illustrated in Fig. 1b , the activity of inverse CeO 2 /Cu catalyst was very close to that of commercial Cu–Zn–Al, approaching the equilibrium in harsh reaction conditions. To further demonstrate the promotion of WGS activity, r values at 300 °C for different catalysts were illustrated in Fig. 1c . Normal Cu/CeO 2 gave r of 10.2 μmol g −1 s −1 , slightly higher than that of reported Cu–Ce(La)O x (9.0 μmol g −1 s −1 ) [15] . The similar r values here reflected the general WGS activity of supported Cu/CeO 2 catalysts. Meanwhile, the inverse CeO 2 /Cu gave a very high r value of 47.3 μmol g −1 s −1 , which was five times that of normal Cu/CeO 2 catalyst. Compared to former inverse CeO x /Cu catalyst (9.8 μmol g −1 s −1 ) [29] , the r of inverse CeO 2 /Cu was also much higher. 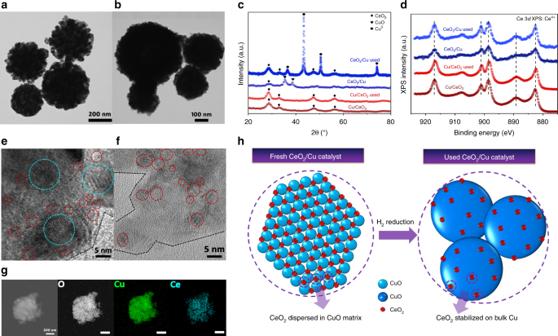Fig. 2 Structure evolution of inverse CeO2/Cu catalyst during WGS reaction.a,bTransmission electron microscope (TEM) images ofafresh andbused inverse CeO2/Cu catalysts.cX-ray diffraction (XRD) patterns of the fresh and used catalysts.dCe 3dX-ray photoelectron spectroscopy (XPS) results of the fresh and used catalysts.e,fHigh-resolution TEM (HR-TEM) images of fresheand usedfinverse CeO2/Cu catalyst, red circles reflect to CeO2, blue circles reflect to CuO.gScanning transmission electron microscope (STEM) image and element mapping results of used inverse CeO2/Cu catalyst, the inset bar: 200 nm.hScheme of structural evolution for inverse CeO2/Cu catalyst during WGS reaction, CeO2nanoparticles are well stabilized despite Cu sintering The activities of some efficient WGS catalysts are listed in Supplementary Table 2 . The inverse CeO x /Cu catalyst exhibited the highest r among the Cu-based catalysts, and its activity was even close to supported Pt catalysts [36] , [37] . Thus, we believe that the inverse CeO 2 /Cu catalyst with tremendous WGS activity has been successively developed. Arrhenius plots for the catalysts were constructed by using the ln of r (Supplementary Fig. 2 ). In the repeated experiments, the WGS on inverse CeO 2 /Cu gave an apparent energy ( E a ) of ca. 37 kJ mol −1 , which was a little lower than that (ca. 40 kJ mol −1 ) found on normal Cu/CeO 2 . Table 1 Physicochemical properties of fresh and used catalysts Full size table Fig. 1 Catalytic performances of the inverse CeO 2 /Cu catalyst. a Water–gas shift (WGS) activities of the inverse CeO 2 /Cu and normal Cu/CeO 2 catalysts. b WGS activities of the inverse CeO 2 /Cu catalyst and commercial Cu–Zn–Al under industrial atmosphere. c Comparison of WGS reaction rates for different catalysts at 300 °C. d Time-on-stream tests of the inverse CeO 2 /Cu, normal Cu/CeO 2 catalysts, and commercial Cu–Zn–Al Full size image For WGS catalysts, sintering is often considered as the main reason for deactivation [8] , [9] , [10] , [38] . The well-dispersed active species may aggregate and deactivate rapidly under reaction conditions. Figure 1d present the results of time-on-stream stability tests. Normal Cu/CeO 2 gave very low r (3 μmol g −1 s −1 ), while the inverse CeO 2 /Cu exhibited surprisingly high stability. With the temperature of 250 °C and very high space velocity of 600,000 cm 3 g −1 h −1 , the WGS r of the inverse CeO 2 /Cu maintained at 17 μmol g −1 s −1 , showing negligible decrease in the test up to 50 h. The long-term stability of commercial Cu–Zn–Al was measured as well. The initial r of Cu–Zn–Al was slightly higher than that of inverse CeO 2 /Cu. After 50 h test, the r dropped from 19.5 to 14.8 μmol g −1 s −1 . Thus, the CeO 2 /Cu catalyst gave very solid performance in the time-on-stream test, which showed superior stability under very high space velocity (600,000 cm 3 g −1 h −1 ). Construction of bulk–nano interfaces The catalytic performances were largely determined by the structure of the catalysts. CeO 2 has been well known as suitable support for Cu catalysts, since the strong interaction between CuO and CeO 2 could achieve homogeneous Cu dispersion [39] , [40] , [41] . For the fresh CeO 2 /Cu catalyst, such interaction could be confirmed by temperature-programmed reduction by H 2 (H 2 -TPR), with the fact that reducibility for CuO was enhanced after CeO 2 addition (Supplementary Fig. 3 ). Moreover, the strong CuO–CeO 2 interaction was convinced by the X-ray photoelectron spectroscopy (XPS) (Supplementary Fig. 4a ) and ultraviolet–visible spectroscopy (UV–vis) analysis (Supplementary Fig. 5a ), showing peak shifting and broadening with increased CeO 2 content. The strong CuO–CeO 2 interaction enhanced the redox properties of the catalysts, and improved the dispersion of both Cu and CeO 2 . Raman spectra of the catalysts depicted in Supplementary Fig. 5b exhibited a tiny peak of Raman mode A g [42] , [43] , which belonged to cupric oxide. Thus, it seemed difficult to tell whether CeO 2 was doped into CuO lattice. The structural and chemical information of inverse CeO 2 /Cu catalyst is given in Fig. 2 . The transmission electron microscopy (TEM) image (Fig. 2a ) of fresh inverse CeO 2 /Cu catalysts present morphology of microspheres with diameters ranging from 200 to 500 nm. These microspheres were stacked of CuO and CeO 2 nanoparticles. After WGS reaction, the microspheres became condensed and formed bulk particles (Fig. 2b ). Catalysts with other Cu–Ce ratios exhibited similar size and morphology (Supplementary Fig. 6 ). Powder X-ray diffraction (XRD) results (Supplementary Fig. 7 ) showed that monoclinic CuO and fluorite CeO 2 served as dominate phase for the fresh catalyst. In Fig. 2c , the XRD pattern of Cu/CeO 2 had no observable change after WGS test, indicating the Cu-species remained well-dispersed. This observation correlated well with the stable nature of Cu/CeO 2 (Fig. 1d ). For inverse CeO 2 /Cu catalyst, sharp metallic Cu peaks emerged after WGS test, and the crystalline size of Cu reached 101.2 nm (Table 1 ). The XRD results were consistent with the trend of dispersity for Cu (Supplementary Table 1 ), though CeO 2 has been found to participate in N 2 O chemisorption, causing higher measured dispersion [44] . The XRD data demonstrated that the CeO 2 /Cu catalyst underwent severe sintering and bulk Cu was formed during WGS reaction. However, even though formation of bulk Cu was observed, the WGS activity and long-term stability of inverse CeO 2 /Cu were surprisingly excellent (Fig. 1 ). This finding was contrary to former knowledge that WGS was favored with smaller Cu-species [38] , [45] . The unusual phenomenon could be well explained by the fact that WGS reaction occurred at CeO 2 –Cu interfaces of inverse CeO 2 /Cu. As the bulk Cu was present, sufficient interfaces could be created if CeO 2 was well dispersed. Small CeO 2 nanoparticles supported on CuO were confirmed by high-resolution TEM (HR-TEM) images in Fig. 2e and Supplementary Fig. 8 . After WGS reaction, small-sized CeO 2 (2–3 nm) was still well-dispersed on bulk Cu (Fig. 2f and Supplementary Fig. 8 ). The element mapping results (Fig. 2g ) further demonstrated the high dispersion of CeO 2 , with Ce signal appearing uniformly on the surface of used CeO 2 /Cu catalyst. XPS profiles of Ce 3 d were recorded in Fig. 2d . For both inverse and normal catalysts, Ce 4+ present as the dominating chemical state before and after WGS reaction. The other prepared Cu–CeO 2 catalysts also exhibited only Ce 4+ (Supplementary Fig. 4b ). Combining with the fact that no shift for the CeO 2 XRD peaks were observed (Fig. 2c ), we believed that the CeO 2 nanoparticles were supported on CuO, rather than incorporated into the CuO lattice. Therefore, enriched CeO 2 –Cu interfaces were present in the inverse CeO 2 /Cu catalyst. Fig. 2 Structure evolution of inverse CeO 2 /Cu catalyst during WGS reaction. a , b Transmission electron microscope (TEM) images of a fresh and b used inverse CeO 2 /Cu catalysts. c X-ray diffraction (XRD) patterns of the fresh and used catalysts. d Ce 3 d X-ray photoelectron spectroscopy (XPS) results of the fresh and used catalysts. e , f High-resolution TEM (HR-TEM) images of fresh e and used f inverse CeO 2 /Cu catalyst, red circles reflect to CeO 2 , blue circles reflect to CuO. g Scanning transmission electron microscope (STEM) image and element mapping results of used inverse CeO 2 /Cu catalyst, the inset bar: 200 nm. h Scheme of structural evolution for inverse CeO 2 /Cu catalyst during WGS reaction, CeO 2 nanoparticles are well stabilized despite Cu sintering Full size image The structural evolution of the inverse catalyst is depicted in Fig. 2h . With the strong interaction, CeO 2 nanoparticles were well dispersed in CuO matrix of the fresh sample. After H 2 reduction, CuO was reduced and sintered to form bulk Cu. Meanwhile, the CeO 2 nanoparticles showed outstanding stability, holding high dispersion under WGS conditions. The aerosol-spray method enabled the inverse CeO 2 /Cu catalyst to give homogeneous Cu–CeO 2 dispersion, which induced an in situ structural transformation, resulting in CeO 2 nanoparticles (2–3 nm) stabilized on bulk Cu. The construction of bulk–nano interfaces brought stable structure of bulk materials and high dispersion of nano-sized catalysts. Tremendous promotion in WGS activity was thus achieved via creation of such bulk–nano interfaces, which was no longer at the risk of sintering deactivation. Simulation of sintering via in situ XRD In order to better simulate the sintering phenomenon during catalysis, in situ XRD measurements under 5% H 2 /Ar were performed towards the inverse and normal catalysts. As shown in Fig. 3a , the peaks for metallic Cu of inverse CeO 2 /Cu catalyst emerged at 150 °C and sharpened, indicating rapid sintering of Cu. Amplified Cu region in Fig. 3d illustrates that bulk Cu formed below 200 °C. For normal Cu/CeO 2 catalyst (Fig. 3b ), no obvious Cu peaks could be observed. Amplified Cu region in Fig. 3e displayed a tiny Cu peak centered at 43°. The Cu peak was absent for used Cu/CeO 2 catalyst (Fig. 2c ), which might due to the re-oxidation and dispersion of Cu under ex situ mode. Besides, the structural evolutions of CeO 2 under reduction are given in Fig. 3c, e . The broad peaks suggested that CeO 2 nanoparticles in inverse CeO 2 /Cu were maintained at very small size (2.1–2.9 nm, Supplementary Fig. 9 ), which was in accordance to the XRD data of used inverse catalyst (2.6–2.7 nm, Table 1 ). 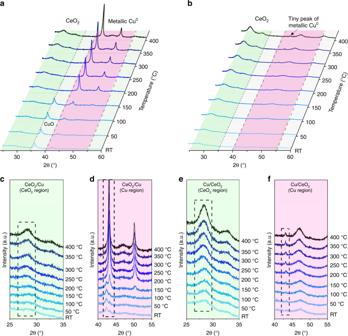Fig. 3 Simulation of sintering via in situ XRD.aIn situ XRD patterns under 5% H2–Ar for inverse CeO2/Cu catalyst.bIn situ XRD patterns under 5% H2–Ar for normal Cu/CeO2catalyst.cAmplified CeO2region of in situ XRD patterns for inverse CeO2/Cu catalyst.dAmplified Cu region of in situ XRD patterns for inverse CeO2/Cu catalyst.eAmplified CeO2region of in situ XRD patterns for normal Cu/CeO2catalyst.fAmplified Cu region of in situ XRD patterns for normal Cu/CeO2catalyst Figure 3e shows that the CeO 2 size of normal Cu/CeO 2 grew under H 2 reduction (2.8–5.3 nm, Supplementary Fig. 9 ). Thus, compared to depositing Cu nanoparticles on CeO 2 support, the dispersion of CeO 2 on bulk Cu created more stable CeO 2 –Cu interfaces. This enrichment of stable interfaces for inverse CeO 2 /Cu catalyst resulted in tremendous promotion of WGS activity, corresponding well to former report, in which Cu–CeO 2 interface was suggested to have great importance in WGS model catalyst [18] . Fig. 3 Simulation of sintering via in situ XRD. a In situ XRD patterns under 5% H 2 –Ar for inverse CeO 2 /Cu catalyst. b In situ XRD patterns under 5% H 2 –Ar for normal Cu/CeO 2 catalyst. c Amplified CeO 2 region of in situ XRD patterns for inverse CeO 2 /Cu catalyst. d Amplified Cu region of in situ XRD patterns for inverse CeO 2 /Cu catalyst. e Amplified CeO 2 region of in situ XRD patterns for normal Cu/CeO 2 catalyst. f Amplified Cu region of in situ XRD patterns for normal Cu/CeO 2 catalyst Full size image WGS mechanism study For WGS reaction, two catalytic mechanisms have been proposed, namely, redox mechanism and associative mechanism [46] , [47] , [48] . In the redox mechanism, CO reacts with surface oxygen of supports after adsorption, forming CO 2 and oxygen vacancy. H 2 O dissociates at the vacancy and produces H 2 . In the associative mechanism, CO and H 2 O adsorb on the catalyst to form an intermediate, which decomposes to yield CO 2 and H 2 . It has been proved that with associative mechanism, surface hydroxyl serves as the active species in Au/CeO 2 system [49] , [50] . In this case, two CO molecules react with two surface hydroxyl groups to form 2 CO 2 molecules and 1 H 2 molecule: 
    2CO + 2OH = 2 CO_2 + H_2
 The amount of produced CO 2 is supposed to be double of that of H 2 in the outlet gas. Temperature-programmed surface reaction (TPSR) were carried out to check the reaction pathway. As shown in Fig. 4b , CO purging gave the ratio of generated CO 2 and H 2 as 2:1, corresponding very well to the above reaction. After H 2 O was introduced, no H 2 signal was detected on Cu/CeO 2 , proving the pure associative mechanism for the normal Cu/CeO 2 catalyst. However, for the inverse CeO 2 /Cu catalyst (Fig. 4a ), the ratio of generated CO 2 and H 2 was 3:1 after CO introduction. This meant that besides the surface hydroxyls, active oxygen atoms created by the dissociation of H 2 O were also involved in the reaction. When H 2 O was injected, H 2 formation could be observed immediately. These observations matched the features of redox mechanism, assuming that H 2 O dissociated on CeO 2 oxygen vacancy to generate H 2 and active surface oxygen atoms. After H 2 O injection, we removed the surface oxygen with H 2 reduction and preserved the surface hydroxyls [50] , after which CO was purged into the system to conduct the TPSR test again. The subsequent CO treatment gave a CO 2 :H 2 ratio of 2:1, showing the typical results of associative mechanism. The TPSR experiment was cycled three times in a row, and it gave very repeatable results for both catalysts. Thus, it turned out that both the redox and associative mechanism were present in the WGS reaction catalyzed by the inverse CeO 2 /Cu catalyst. Fig. 4 WGS mechanism study of the inverse CeO 2 /Cu catalyst. a Temperature-programmed surface reaction (TPSR) on the inverse CeO 2 /Cu with consecutive switch of CO, H 2 O, and H 2 at 200 °C. b TPSR on normal Cu/CeO 2 with consecutive switch of CO, H 2 O, and H 2 at 200 °C. c Temperature-programmed desorption of CO (CO-TPD) and d in situ diffused reflectance infrared Fourier transform spectroscopy (DRIFTS) results of the inverse CeO 2 /Cu under the WGS conditions (2%CO/2%H 2 O/Ar, at 200 °C) Full size image It has been generally believed that the redox mechanism occurs on metals [46] , [47] and the associative mechanism dominates at the metal/oxide interface [50] , [51] . However, redox pathway has now been found on inverse CeO 2 /Cu catalyst. The improved redox properties of CeO 2 nanoparticles on inverse CeO 2 /Cu played an important role. Temperature-programmed desorption of CO (CO-TPD) was applied to detect the CO sorption on the inverse catalyst. As illustrated in Fig. 4c , after CO pre-adsorption, CO 2 was the only desorption species on CeO 2 /Cu, showing easy transformation from CO to CO 2 . For better study over CO adsorption, diffuse reflectance infrared Fourier transform spectroscopy (DRIFTS) was introduced. As shown in Fig. 4d , the in situ DRIFTS of the inverse CeO 2 /Cu catalyst under WGS conditions exhibited CO 2 signal [52] (2334, 2364 cm −1 ) at the beginning, which indicated the ongoing of WGS reaction. Meanwhile, no signal of CO was detected during the measurement, while normal Cu/CeO 2 gave CO–Cu 0 adsorption (2094 cm −1 ) [53] , [54] (Supplementary Fig. 10b ). Pure Cu showed no adsorption behavior under both WGS and CO modes, suggesting CO adsorption on bulk Cu was not favored (Supplementary Fig. 10c and d ). Besides, the results of in situ DRIFTS for CO adsorption on the CeO 2 /Cu also only present CO 2 signal, which showed that active surface species of the catalyst was reduced by CO (Supplementary Fig. 10a ). Besides, we measured the reaction orders of CO and H 2 O for different catalysts. As shown in Supplementary Fig. 11 , the H 2 O reaction order increased when CeO 2 content was elevated, giving the catalyst stronger capability to consume H 2 O. The CO reaction order on inverse CeO 2 /Cu was 0.75, which suggested CO was comparatively insufficient during WGS reaction. All the above data demonstrated the easy transformation from CO to CO 2 on inverse CeO 2 /Cu, reflecting unique redox properties of the CeO 2 nanoparticles. The surface oxygen of inverse CeO 2 /Cu was proved to be flexible under CO, which facilitated the formation of defect sites. Role of the surface defects in the catalysts The formation of defect sites on inverse CeO 2 /Cu were evidenced by in situ Raman measurements, since ex situ Raman and XPS results did not show pronounced Ce 3+ signals. As shown in Fig. 5a , the Raman spectra of the inverse CeO 2 /Cu after H 2 activation gave a hump at 600 cm −1 , which was ascribed to the intrinsic defects [55] , [56] . When CO was filled in, surface oxygen was removed, forming two characteristic peaks located at 546 and 456 cm −1 , respectively. The peak centered at 546 cm −1 ( D peak) resulted from defects where Ce 4+ was replaced by Ce 3+ [56] , and the peak centered at 456 cm −1 was typical vibration mode ( F 2g ) of fluorite-type structure [56] , [57] . It is surprising that the Raman signals of the inverse CeO 2 /Cu showed that the defect D peak was even more pronounced than F 2g peak. When H 2 O was introduced, the intensity of the D peaks decreased apparently, which meant the Ce 3+ defects were filled. The second cycle gave the same results. The introduction of CO induced the creation of surface defects through the reaction: 
    CO + O→CO_2
 
    CO + OH→CO_2 + 1/2H_2
 Fig. 5 Examination of defect sites in the catalysts. a In situ Raman spectra of the inverse CeO 2 /Cu with CO/H 2 O switch under 200 °C. b In situ Raman spectra of the normal Cu/CeO 2 with CO/H 2 O switch under 200 °C. c In situ Raman under the WGS conditions for both catalysts, the inset figure gave D / F 2g integral ratio at different temperatures Full size image For the normal Cu/CeO 2 catalyst (Fig. 5b ), the intensity of Ce 3+ D peaks was clearly weakened. The generation and elimination of defects with the CO/H 2 O switch was also sluggish. In situ Raman under WGS conditions (Fig. 5c ) showed consistent results. The inverse CeO 2 /Cu also gave more pronounced signal of surface defects under the WGS conditions, with D / F 2g integral ratio of 1.8. These results were totally different from those of pure CeO 2 sample (Supplementary Fig. 12 ), which gave very strong F 2g peak and nearly no defect peak. The in situ Raman results have confirmed the enrichment of Ce 3+ defect sites in inverse CeO 2 /Cu under WGS conditions, which further proved the enhanced redox properties of CeO 2 on inverse CeO 2 /Cu. For both catalysts, metallic Cu was the only phase detected under the WGS conditions. Supplementary Fig. 13 displayed the TPSR results of inverse CeO 2 /Cu and normal Cu/CeO 2 catalysts. The WGS reaction began to occur at ~100 °C. After TPSR, the following H 2 -TPR measurement gave no H 2 reduction peaks, which suggested Cu remained in fully metallic state during the WGS reaction. This finding was in accordance with the former work reported by Barrio et al. [29] However, considering the very high WGS activity of the inverse CeO 2 /Cu catalyst, the active site was more likely to locate at Cu–CeO 2 interfaces rather than metallic Cu. The mixed oxides of Cu–Zn–Al have been applied as industrial WGS catalysts for decades. Though lots of efforts have been made, few reports have found Cu-based catalysts as effective as Cu–Zn–Al, especially under industrial atmosphere. 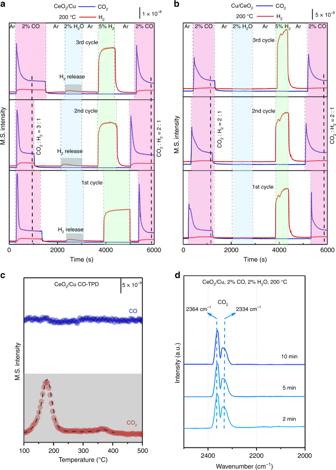Fig. 4 WGS mechanism study of the inverse CeO2/Cu catalyst.aTemperature-programmed surface reaction (TPSR) on the inverse CeO2/Cu with consecutive switch of CO, H2O, and H2at 200 °C.bTPSR on normal Cu/CeO2with consecutive switch of CO, H2O, and H2at 200 °C.cTemperature-programmed desorption of CO (CO-TPD) anddin situ diffused reflectance infrared Fourier transform spectroscopy (DRIFTS) results of the inverse CeO2/Cu under the WGS conditions (2%CO/2%H2O/Ar, at 200 °C) Herein, the inverse CeO 2 /Cu catalyst showed greatly promoted WGS activity, which was five times higher than that of normal Cu/CeO 2 catalyst. The WGS conversion of the inverse CeO 2 /Cu was very close to that of commercial Cu–Zn–Al under industrial WGS atmosphere, approaching the equilibrium maximum. The high WGS activity for the inverse CeO 2 /Cu catalyst originated from its unique structure, where bulk–nano interfaces were constructed. When Cu was loaded on CeO 2 , sintering was inevitable as the aggregation of Cu species lowered the surface energy. The dynamic elimination of Cu–CeO 2 interfaces caused rapid deactivation. Thus, for normal Cu/CeO 2 catalyst, though Cu–CeO 2 interfaces were created, the elimination due to structural change would take place even in H 2 pre-treatment. This deactivation resulted in very low WGS r in activity and stability tests (Fig. 1a, d ). Considering its high Cu dispersion, the turnover frequency (TOF) of normal Cu/CeO 2 was calculated for single site on Cu–CeO 2 interface (see detail in Supplementary Methods ). The derived TOF was 0.056 s −1 , as shown in Table 1 . Meanwhile, for inverse CeO 2 /Cu catalyst, bulk Cu formed steady structure under WGS conditions. Small CeO 2 nanoparticles were dispersed on bulk Cu and were also very stable against sintering. The maximized and stabilized bulk–nano interfaces in the inverse CeO 2 /Cu catalyst gave significant WGS promotion. The high WGS activity resulted from the structural nature of the inverse CeO 2 /Cu catalyst, which lied in creation and preservation of stabilized bulk–nano interfaces. A theoretical model has been built to calculate TOF for the inverse CeO 2 /Cu. A 3 nm CeO 2 nanoparticle with 231 Ce atoms was loaded on metallic Cu. As shown in Supplementary Fig. 14 , 16 Ce atoms were located at the periphery of Cu–CeO 2 interface. Based on this model, the TOF of the inverse CeO 2 /Cu catalyst for single site on CeO 2 –Cu interface was 0.058 s −1 (see detail in Supplementary Methods ). The similar TOF of both catalysts proved that the Cu–CeO 2 and CeO 2 –Cu interfaces possessed the same intrinsic activities. As shown in Table 1 , the amount of interface sites for inverse CeO 2 /Cu was four times higher than that for normal Cu/CeO 2 . The highly promoted WGS activity of inverse CeO 2 /Cu originated from the enrichment of interface sites. Besides, owing to the strong Cu–CeO 2 interaction, the redox properties of inverse CeO 2 /Cu catalyst were improved. The surface oxygen of inverse CeO 2 /Cu catalyst was proved to be flexible under CO, leading to the formation of defects. H 2 O dissociated at the defects, promoting the WGS activity via a combination of both the associative mechanism and redox mechanism. The discussion of reactivity and mechanism was concluded in Fig. 6 . Fig. 6 Role of inverse CeO 2 /Cu in catalyzing the WGS reaction. Role of the CeO 2 –Cu interfaces in catalyzing the WGS reaction on inverse CeO 2 /Cu catalyst Full size image The pursuing of highly active and stable catalysts would never be out of date. A strategy to fabricate robust WGS catalyst was proposed, where the key was the construction of bulk–nano interfaces. By using aerosol-spray method, we developed the CeO 2 /Cu catalysts with inverse configuration. Small CeO 2 nanoparticles (2–3 nm) were stabilized on bulk Cu, forming stable CeO 2 –Cu interfaces under reaction conditions. The enrichment and preservation of such interfaces resulted in significant promotion in activity. The inverse CeO 2 /Cu catalyst exhibited great WGS activity, which was at least five times higher than other reported Cu catalysts. The improved redox properties of the inverse CeO 2 /Cu catalyst facilitated the H 2 O dissociation and CO oxidation, boosting WGS activity via the combination of associative and redox mechanism. Catalyst with sufficient bulk–nano interfaces has now been proved to give excellent WGS performances under realistic conditions, and show great potentials in practical applications and other catalytic systems. Catalyst preparation In a typical synthesis of Cu a Ce b O x , 4 mmol of metal nitrates (99%, Tianjin Kermal Factory) were added to 60 ml of absolute ethanol (99%, Tianjin Fuyu Fine Chemical Reagent Factory). This mixture was stirred for 10 min and then put into a ultrasonic humidifier (30 W, 1.5 MHz). Industrial N 2 served as the carrier gas to bring the spray generated through sonication into the tube furnace (pre-heated to 400 °C). The mist drop evaporated and the precursor underwent decomposition and self-assembly. The metal oxides products were spherical nanoparticles, which were collected on a piece of filter paper and dried overnight at 60 °C. Then, the obtained powder was calcined in air for 4 h (1 °C min −1 of ramping rate). The obtained catalysts were nominated as Cu a Ce b O x , of which a and b referred to the molar ratio of corresponding element, respectively. Commercial Cu–Zn–Al catalyst (37 wt% CuO, 52 wt% ZnO, 11 wt% Al 2 O 3 , determined by EDS) was bought from Sichuan Shutai Chemical Engineering Company. Transmission electron microscope (TEM) All images of TEM were taken on a JEOL JEM-2100F microscope, of which the acceleration voltage was 200 kV. The images of HR-TEM were obtained by using a Philips Tecnai F20 instrument with the acceleration voltage of 200 kV. The element mapping results and EDS analysis were acquired from the same machine under STEM mode. X-ray diffraction (XRD) For the XRD data, all experiments were performed on a PANalytical B.V. X’pert3 powder diffractometer with CuK α radiation ( λ = 0.15418 nm). Accelerating voltage and current of 40 kV and 40 mA were applied for ex situ and in situ modes. Ex situ XRD patterns were obtained by using a PIXcell D detector in the 2 θ range of 20‒80°. For the in situ XRD experiments, an Anton Paar XRK900 in situ chamber was applied. The XRD data were measured from 50 to 400 °C in 5% H 2 /Ar mixture (30 cm 3 min −1 ). X-ray photoelectron spectroscopy (XPS) The XPS measurements were performed on an Axis Ultra XPS spectrometer from Kratos, Japan. The operation was under 225 W of accelerating voltage and Al K α radiation. The C 1 s line located at 284.8 eV was used to calibrate each spectra for accurate binding energies. Raman spectroscopy Ex situ and in situ Raman spectra were obtained by excitation of the catalysts at 633 nm laser, using a LabRAM HR800 Raman spectrometer (Horiba Jobin Yvon) with the range from 200 to 800 cm −1 in a spectral resolution of 2 cm −1 . Temperature-programmed surface reaction (TPSR) An online mass spectrometer (Ametek LC-D200M) was used to analyze the outlet gases for TPSR, as well as CO-TPD. 100 mg of each sample were treated with 5% H 2 /Ar (30 cm 3 min −1 ) for 30 min at 300 °C before test. The sample was then flushed under pure He for 1 h. For CO-TPD, the samples were purged with 5% CO/Ar (30 cm 3 min −1 ) for 0.5 h, and then flushed under pure He for another 1 h at room temperature. Afterwards, the samples were heated from room temperature to 500 °C under He flow. For TPSR, the catalysts were heated from 120 to 400 °C under 2%H 2 O, 2% CO/Ar gas flow (30 cm 3 min −1 ). For the examination of reaction mechanisms, the samples went through WGS reaction for 1 h at 200 °C after H 2 reduction. 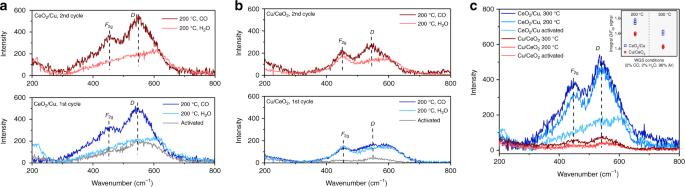Fig. 5 Examination of defect sites in the catalysts.aIn situ Raman spectra of the inverse CeO2/Cu with CO/H2O switch under 200 °C.bIn situ Raman spectra of the normal Cu/CeO2with CO/H2O switch under 200 °C.cIn situ Raman under the WGS conditions for both catalysts, the inset figure gaveD/F2gintegral ratio at different temperatures 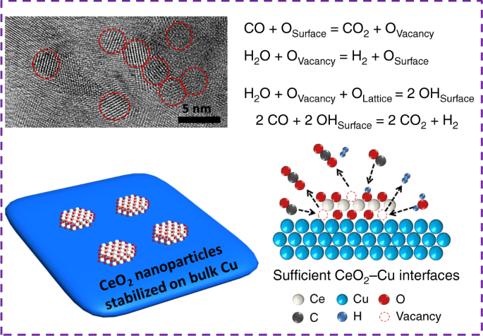Fig. 6 Role of inverse CeO2/Cu in catalyzing the WGS reaction. Role of the CeO2–Cu interfaces in catalyzing the WGS reaction on inverse CeO2/Cu catalyst The catalysts were then purged by Ar at 200 °C, followed by the switch of 2%CO/Ar, pure Ar, 2%H 2 O/Ar, pure Ar, 5%H 2 /Ar, pure Ar, and 2%CO/Ar to collect the mass spectrometer signal. The heating rate for all tests was set as 10 °C min −1 . Catalytic tests and kinetics measurement A fixed-bed reactor with diameter of 1 cm was used for the WGS reaction tests. In order to give accurate results, a thermocouple connected with a PID temperature controller was mounted on top of the catalyst bed. The catalyst powder (100 mg) was loaded and reduced with 5% H 2 /Ar mixture for 0.5 h at 300 °C. The reaction gas contained 2% CO and 10% H 2 O, balanced with N 2 . The total gas hourly space velocity (GHSV) was 42,000 cm 3 g −1 h −1 . In order to prevent water condensation, all pipes of the reactor were binded with heating belts. The activity results of catalysts were measured from 150 to 400 °C as 50 °C per step. Each catalyst was tested repeatedly to rule out the uncertainty. A Gasboard 3500 IR spectroscopy (WuhanSifang Company, China) was used to analyze all the outlet gases online. For the stability tests, the CO conversion data of the catalysts were continuously recorded under 250 °C for 50 h. The mass of the catalysts and the flow rate of reaction gas were tuned to keep the CO conversion under 15%. The WGS activity was measured by means of CO conversion, which was defined as the following formula: 
    X_CO( %) = ( n_CO^in - n_CO^out)/n_CO^in×100%
 (1) For the kinetic tests, 20 mg of catalysts were pre-reduced with 5% H 2 /Ar mixture. The apparent activation energy ( E a ) of each catalyst for WGS reaction was obtained by keeping 10% equal CO conversion with the regulation of reaction temperature, catalysts mass, and stream flow rate. The calculation of reaction rate ( r ) for WGS followed the equation: 
    r = F ×CO_converted/W
 (2) where F is the total flow rate of the reaction stream (mol s −1 ). r is the WGS reaction rate by means of CO (mol g −1 s −1 ). CO converted is the concentration of converted CO on the IR spectroscopy and W is the mass of the catalyst (g). The reaction orders of CO and H 2 O for the catalysts were measured under 250 °C. The WGS activity was recorded while the concentration of CO or H 2 O in the reaction gas was varied on purpose.